Perturbative optical parametric amplification in the extreme ultraviolet The response of a medium illuminated with a light field can be expanded in many orders in perturbative non-linear optics. Here we use two multiple-cycle high-intensity laser pulses at 800 and 1,400 nm to generate extreme ultraviolet radiation where the multi-photon processes can be treated as the driving force of a perturbative optical parametric amplification. When a very high-intensity pulse (>7.10 14 W cm −2 ) at 800 nm is applied in addition to a high-intensity pulse at 1,400 nm, we are able to enhance the flux of the coherent extreme ultraviolet radiation in the photon energy range around 80 eV by more than an order of magnitude compared with the generation with a single-wavelength pulse. This opens the way to extend the powerful techniques of perturbative non-linear optics to the case of a high-intensity-driving field in multiple-photon processes. The response of a medium illuminated by a light field can be described by perturbative or non-perturbative non-linear optics that are conceptually very different. In perturbative non-linear optics [1] , the response of the medium is expanded in many orders, expressed as linear and non-linear terms in which high orders of response are taken into account. In non-perturbative non-linear optics, the light interaction with the medium can be approximated by a classical or quantum treatment through the time-dependent Schrödinger equation. Various schemes for the generation of coherent soft X-ray and X-ray radiation have been demonstrated, such as high-order harmonic generation (HHG), soft X-ray free-electron lasers and plasma-based X-ray lasers based on the acceleration of free electrons. The non-perturbative treatment has been used in the three-step model for HHG [2] , where an electron is first liberated from an atom through strong field ionization, then accelerated by the laser field and finally recombined with the parent ion, emitting any excess energy as a high-energy photon. The photon flux, coherence and beam quality of the output radiation are very different for the various schemes and depend on the configuration for the X-ray generation. The low coherence properties of the radiation from X-ray free-electron lasers and soft X-ray lasers radiation can be improved by seeding with coherent high-harmonic radiation [3] , [4] . To obtain high-intensity radiation, Seres et al . [5] , [6] suggested parametric stimulated soft X-ray emission in which the gain is obtained by accelerating electrons with the strongly non-linear Coulomb field of ions in a gaseous medium. The Coulomb field of the ion plays an important role in the recombination of the free electron with its parent ion. Bertrand et al . [7] have recently shown that when two intense fundamental laser pulses of frequency ω 1 and ω 2 are crossed non-collinearly in a gas-jet target, the HHG spectrum can be described simply in terms of conservation of energy and momentum based on the net number of photons absorbed from each laser field. The observation of non-linear optical wave mixing in HHG [7] also suggests the possibility to construct a perturbative non-linear optics theory for the physics of HHG. On the basis of perturbative non-linear optics, Meye et al . [8] , [9] have proposed a high-order parametric amplifier for generating radiation in the extreme ultraviolet (XUV) region where the signal ( ω s ) and idler ( ω i ) waves are generated by a multi-photon process qω p = ω s + ω i . However, this process has not been clearly realized in experiments. In this paper, we report the generation of XUV radiation by the optical parametric amplification process. In comparison with the generation of XUV radiation using a single pulse at 1400, nm (or 800 nm), a remarkable enhancement of the flux of the coherent XUV radiation in the photon energy range around 80 eV, together with numerous spectral components in a large bandwidth of 35 eV, is obtained by pumping with an additional 800-nm high-intensity multiple-cycle pulse. This opens the way to extend the powerful techniques of perturbative non-linear optics to the case of a high-intensity-driving field in multiple-photon processes. High-order harmonic generation An ∼ 30-mm-long cell filled with argon gas at a pressure of up to 500 Torr is used as the interaction medium [10] , [11] . The high-order harmonic radiation can be generated at wavelengths down to 16 nm when an 800 nm pulse, a 1,400-nm pulse or both pulses together are applied (see Methods section—Experimental arrangement). When only the 1,400-nm pulse ( ∼ 2.10 14 W cm −2 ) is applied as the driving pulse, we can obtain phase-matched HHG radiation [11] with well-resolved odd harmonics (green dashed line in Fig. 1 and Supplementary Fig. 1 ) and a good beam profile along the propagation direction of the driving pulse. The total HHG intensity is a maximum when the focus of the 1,400-nm beam is ∼ 1 mm inside the gas cell. The spectrum of the HHG radiation generated by the intense 800-nm driving pulse is complex—not only odd orders but also even orders and non-integer orders are generated (red dashed line in Fig. 1 ) and the beam profile is broad. The intensity of radiation <20 nm is very weak. Without considering the defocusing caused by the plasma, the intensity of the 800-nm pulse is estimated to be >7.10 14 W cm −2 around the focus and the ionization fraction is >50% at the peak of the pump pulse, which is much larger than the critical ionization fraction (<3%) for the phase-matched generation of high-order harmonics in an argon medium [12] . The generation of weak harmonics in the wavelength range around 20 nm with the 800-nm beam confirms that the strength of the high-order non-linearity created by the 800-nm field is large enough to drive multiple-photon processes. 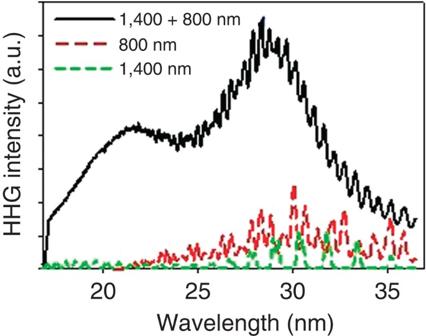Figure 1: Spectrum of XUVs. Spectrum of XUV generated by 800 nm (red long dashed line), 1,400 nm pulses (green short dashed line) and both pulses (black solid line) overlapped in time. The inset shows the principle of the parametric amplification. Figure 1: Spectrum of XUVs. Spectrum of XUV generated by 800 nm (red long dashed line), 1,400 nm pulses (green short dashed line) and both pulses (black solid line) overlapped in time. The inset shows the principle of the parametric amplification. Full size image High-order harmonic amplification When the 1,400- and 800-nm pulses are overlapped, that is, for zero time delay (black line in Fig. 1 ), the intensity of the XUV radiation is much higher (by more than an order of magnitude) In this case, XUV radiation with numerous spectral components is obtained. In the non-perturbative three-step model of HHG [2] , the atomic dipole phase is acquired by the electron wave function in the continuum due to the delay between the ionization and recombination times. Depending on the time of ionization of the electron, the contributions of different electron trajectories or different so-called quantum pathways must be considered in the harmonic generation process. The harmonic spectrum exhibits strong shifting and splitting because of the harmonic phase-modulation effect ( Supplementary Note 1 ). This indicates that other mixing processes of the two fields [7] need to be considered and the symmetry of the total field and the atomic system is broken [13] . A minimum in the spectrum can be seen at ∼ 24 nm (51 eV) where a Cooper minimum caused by destructive interference of the 5 s and 4 d transition dipole moments in argon is expected [14] . The observation of a Cooper minimum in the amplified spectrum indicates that a combination of single-atom responses in the non-linear atomic dipole moment can be used in a theoretical treatment. The short wavelength part (<17 nm) is not shown in this figure because of strong absorption by the absorption edge of the aluminium foil. 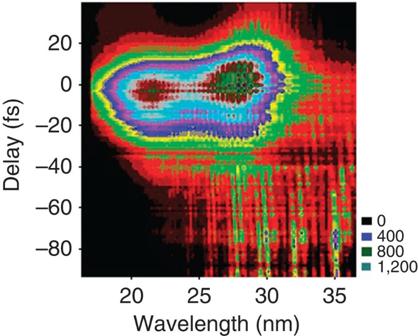Figure 2: Variation of delay time of two pulses. Spectrum of XUV radiation along the optical axis of the pump pulse versus delay time between the 800- and 1,400-nm pulses. HHG intensity and spectrum versus delay time Figure 2 shows the variation of the XUV output spectrum along the propagation direction of the driving laser pulse versus delay time between the two pulses at 800 and 1,400 nm. Positive delay time implies that the 800-nm pulse precedes the 1,400-nm pulse. The position of the focus of the 800 and 1,400 nm beams is located at the exit pinhole and ∼ 1 mm before the exit pinhole, respectively, for a gas pressure of 300 Torr. A maximum of the XUV radiation is obtained when the two pulses are overlapped in time (zero delay). For negative delay, not only the harmonic intensity increases with shorter delay time but also the spectrum of the harmonics changes. When the interaction of the 800-nm pulse is very weak or absent (for negative delay >−80 fs), the harmonic spectrum consists of odd harmonic orders of the 1,400-nm pulse, as expected. For a negative delay time of <−40 fs, other peaks can be seen between the odd orders of 1,400 nm, which are caused by frequency mixing with the 800-nm pulse [7] . A similar effect is observed when the intensity of the 800-nm pulse is weak as shown in Supplementary Fig. 2 and Supplementary Fig. 3 . Around zero-delay time a rich pattern spectrum is detected. The harmonic intensity decreases more rapidly on the positive delay side than on the negative delay side. This is caused by the high ionization rate created by the leading edge of the pump pulse, which increases the phase mismatch. The generation of a visible idler pulse with a different combination of frequency mixing of the two laser pulses m / λ 1 ± n / λ 2 ( λ 1 =800 nm, λ 2 =1,400 nm, where m + n is odd) is observed, which varies with the delay of the two pulses, as shown in Supplementary Fig. 4 and Supplementary Table 1 . Figure 2: Variation of delay time of two pulses. Spectrum of XUV radiation along the optical axis of the pump pulse versus delay time between the 800- and 1,400-nm pulses. Full size image Variation of intensity of the 800-nm pump field To study the dependence of the XUV output radiation on the 800-nm pump field, the two pulses are overlapped in time, that is, the delay time is set to zero. The intensity of the 800-nm pump pulse is varied, while other parameters such as the intensity of the 1,400-nm pulse, the focus position of the two beams and the gas pressure are fixed. The result is displayed in Fig. 3 . A complex spectrum is obtained even at low pump intensity because a weak pump field can modify the trajectory of the free electron created by the 1,400-nm pulse [13] . When the intensity of the pump beam is low, the amplification is small. With high pump intensity (>3 mJ pulse energy), the ionization rate of the gas is high and the phase mismatch increases, and therefore the amplification saturates. A high pump intensity is required, and the saturation is less for the short wavelength part ( ∼ 20 nm) as shown in Fig. 3 . 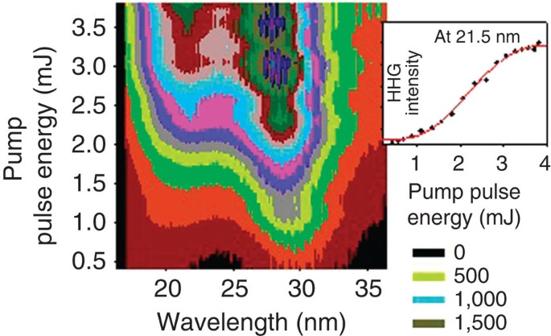Figure 3: Amplified intensity of XUV at different pump intensities. Intensity of XUV radiation versus intensity of the 800 nm pump field with the 800- and 1,400-nm pulses overlapped in time. The inset shows the variation of XUV intensity at 21.5 nm. Figure 3: Amplified intensity of XUV at different pump intensities. Intensity of XUV radiation versus intensity of the 800 nm pump field with the 800- and 1,400-nm pulses overlapped in time. The inset shows the variation of XUV intensity at 21.5 nm. Full size image For a detailed analysis of the dependence of the HHG intensity on the amplification conditions, we consider the intensity of the narrow bandwidth XUV radiation at 21.5 nm, which is shown in the inset of Fig. 3 . The output intensity of the XUV radiation at 21.5 nm can be fitted with equation (9) in Methods (solid line in inset of Fig. 3 ) by considering the phase mismatch dependence on laser intensity using equation (12). In this fit, we consider that the non-linear coupling coefficient γ or the non-linear atomic dipole moment scales as I 3 (ref. 15 ). Variation of interaction length and gas pressure To study the variation of the output XUV radiation versus the interaction length, the focus position of the two beams is varied relative to the exit pinhole of the gas cell. The results are displayed in Fig. 4 where the focus position is taken to be negative (positive) when the focus is outside (inside) the gas cell. When the focus position of the two pulses is located deeper inside the gas cell, the HHG intensity decreases rapidly because of absorption and the large phase mismatch especially in the wavelength range >30 nm. A maximum total XUV intensity is obtained when the focus is located 0.5 mm inside the gas cell. 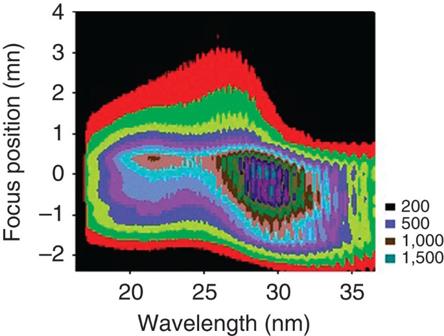Figure 4: Variation of interaction lengths. XUV radiation versus focus position of the 800-nm pulse with the 800- and 1,400-nm pulses overlapped in time. Figure 4: Variation of interaction lengths. XUV radiation versus focus position of the 800-nm pulse with the 800- and 1,400-nm pulses overlapped in time. Full size image Because the dependence of the phase mismatch term on the gas density ( N ) or gas pressure is complex, the phase mismatch term (equation (11) in Methods) can be expanded with equation (12), where x is the pressure. A study of the pressure dependence of the XUV radiation helps to reveal the difference between the amplification and the phase-matched generation process through equations (9) and (13). 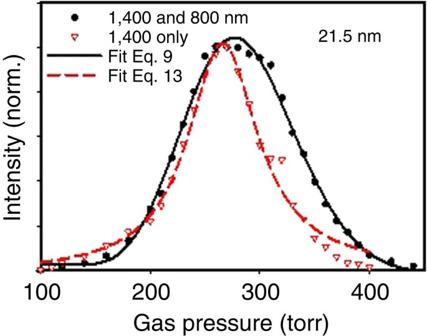Figure 5: Variation of gas pressure. Pressure dependence of the normalized intensity of XUV radiation at 21.5 nm for the case when the two pulses, 800 and 1,400 nm, are applied for amplification (black circles) and when only the 1,400-nm pulse is applied for phase-matched generation (red triangles). Eq., equation; Norm., normalized. Figure 5 shows the variation of harmonic intensity for different pressures (100 to 450 Torr) of the medium. At low gas pressure, the XUV radiation scales as N 2 when the harmonic generation process is phase matched (Δ k ∼ 0) for the 1,400-nm beam. At high pressure, the XUV intensity decreases because of the strong phase mismatch and absorption by the medium, which plays an important role at pressures >350 Torr. When one beam, at 1,400 nm, is applied, the fit using equation (13) is not good for high pressures because of the strong influence of absorption. When the two beams, at 800 and 1,400 nm, are applied, a good fit to the experimental data is obtained with equation (9), as shown by the solid line in Fig. 5 . The measured yield increases exponentially with pressure in the range 150–250 Torr (Δ k ∼ 0), which reflects the amplification process. The phase-mismatch causes a decrease of the XUV intensity in the parametric amplifier, as expected, and is large at high pressure. We note that in the case of two beams present, the fit with equation (13) (see Supplementary Fig. 6 ) is not good at low and high pressure when only phase matching or propagation of the harmonic and fundamental fields is considered [9] , [16] . With the amplification model, we are able not only to account for the XUV intensity but also to determine pump laser parameters such as the pump intensity and interaction length necessary for maximizing the gain. Figure 5: Variation of gas pressure. Pressure dependence of the normalized intensity of XUV radiation at 21.5 nm for the case when the two pulses, 800 and 1,400 nm, are applied for amplification (black circles) and when only the 1,400-nm pulse is applied for phase-matched generation (red triangles). Eq., equation; Norm., normalized. Full size image When the two pulses are overlapped in time, not only the maximum intensity of the harmonic is reached but also the diameter of the XUV beam is smaller ( Supplementary Fig. 7 and Supplementary Fig. 8 ). The good beam profile indicates a high degree of coherence of the XUV beam along the axis of the pump beam. We have realized the concept of perturbative optical parametric amplification for the generation of high flux, highly coherent XUV radiation. We have shown that the presence of amplification accounts for the output of the emission. We also confirm that a perturbative formalism can be developed around the amplification process, up to ultra-high orders of non-linearity, even though the HHG is a highly non-perturbative process. This result is important for the application of infrared (IR) and near-IR-driving pulses for the generation of high-order harmonic radiation and in strong field physics. When an IR-driving pulse is used for generating high-order harmonics, high photon energy radiation is generated but the efficiency is usually low because of quantum diffusion. Parametric amplification can be used to enhance the efficiency. In addition, our amplification provides a high-intensity coherent XUV source with rich spectral components, which can be used for spectroscopic applications in this region or as a seeding pulse in free electron lasers. When a carrier-envelope phase-stabilized high-intensity pulse is applied, the generation of high-intensity attosecond pulses can be realized. Perturbative optical parametric amplification With the consideration of second- and third-order non-linearity, optical parametric generation and optical parametric amplification play an important role in the generation of ultrashort laser pulses in the IR and visible range [17] . The generation and amplification of the new fields is based on the coupling of the signal ( s ) and idler ( i ) fields driven by a strong pump ( p ) field in a non-linear medium. When the pump field with carrier frequency ω p is very strong (>10 7 V cm −1 ), high non-linear orders of the medium response need to be considered. The generation and propagation of the idler and signal fields driven by a high-order non-linear response to the pump field A p can be written [8] , [9] where A j are the amplitudes of the corresponding fields E j ={ A j exp [ i ( k j z + ω j t )]+c.c. }/2, n j are the refractive indices, N is the atomic density, Δ k = qk p −k s −k i is the wavevector mismatch, χ (q+1) ( ω i ) and χ (q+1) ( ω s ) are the ( q+ 1) th non-linear susceptibilities and α i , α s are the absorption coefficients. The general solutions of equations (1) and (2) are where γ is the non-linear coupling coefficient between the idler and signal field. The γ s,i are determined by the amplitudes of the corresponding non-linear atomic dipole moments, which depend on the intensity of the driving field A p and the optical properties of the medium. When ω i is in the visible or IR regions, the absorption by the gas medium is very small, or α i =0 and ω s >> ω i . Experiments and theory of HHG show that the intensity of successively higher harmonic orders does not decrease significantly, as is expected in perturbative non-linear optics. We consider that the non-linear response in equations (1) and (2) is constant over a range of high orders. From quantum mechanical considerations and averaged over quantum interferences, the non-linear atomic dipole moment scales as I 3 , where I is the intensity of the driving field [15] , and then we can consider that | γ| 2 scales as I 3 over a wide range of high orders. When A s0 ≠0 and A i0 =0 are boundary conditions at z =0, the signal field is given by When the non-linear coupling is small ( γ << β ) The intensity of the XUV radiation is then given by Phase mismatch Since the non-linear coupling coefficient γ is small for high-order processes, for the realization of parametric amplification fulfilment of the phase-matching condition, Δ k ≅ 0, is an important requirement and is a rather complex problem in the case of high-intensity laser fields. Energy and momentum conservation are given by qω p = ω s + ω i and q k p = k s + k i . The dispersion of the medium leads to a phase mismatch Δ k =( q k p − k i )− k s ≅ q k p − k s ( q >>1) when the idler field is in the visible or IR regions (as shown in the inset of Fig. 1 ). For a collinear configuration of amplification along the propagation direction ( z ) of the pump field, the phase mismatch without consideration of the phase change of the field around the focus can be written as [18] where λ p is the centre wavelength of the pump pulse, N a is the number density of atoms at 1 atmosphere, η ( t ) is the ionization fraction, r e is the classical electron radius and δn is the difference between the refractive indices, including the non-linear components, at the pump and harmonic wavelengths. The first term in equation (11) is related to the dispersion of the neutral medium, which is negative, and the second term is the plasma dispersion, which is positive. The major sources of phase mismatch are pressure dependent, which allows the phase-matching condition to be satisfied in plasmas with arbitrary electron density. Full phase matching can be achieved within a few optical cycles of the laser pulse by eliminating the phase mismatch. The phase mismatch Δ k is a function of the atomic density (pressure p ), the interaction length ( l ) and the intensity of the pump pulse ( I ) and can be expanded in the form where x represents p , l or I . When a single intense laser field is used for generation of the HHG, the intensity of the phase-matched XUV radiation in a dispersive and absorbing medium is given by [9] where N is the gas density and l is the length of the interaction medium. Experimental arrangement A 1-kHz multi-stage, multi-pass, chirped-pulse Ti:sapphire amplifier system that produces pulses up to 10 mJ with a duration of 30 fs and centred at 800 nm is used for our experiment. The 800-nm laser beam is split into two beams, with pulse energies of 5 and 4 mJ. The 5-mJ beam is used for pumping a standard optical parametric amplifier system to generate an IR pulse at 1,400 nm with an energy of ∼ 1.5 mJ and duration of 40 fs. The 4-mJ beam is used to pump the high-order parametric amplification. Details of the HHG set-up and the detection system have been published elsewhere [10] , [11] . The 1,400-nm IR pulse is used to generate a seed XUV pulse and the 4-mJ pulse at 800 nm is aligned in a co-propagating direction by a dichroic mirror and acts as the pump pulse for amplification. The focus position of the two beams can be varied and shifted relative to each other, which allows control of the intensity of the output XUV radiation. The laser beams are used to drill an exit pinhole in a thin Al plate allowing straightforward handling, and no further alignment procedure along the optical axis is needed. The diameter of the two beams at the focus is ∼ 100 μm. Enhancement of the ionization and Rayleigh scattering from free electrons in the region where the two pulses overlap are used for spatial and temporal alignment of the pulses. How to cite this article: Dao, L.V. et al . Perturbative optical parametric amplification in the extreme ultraviolet. Nat. Commun. 6:7175 doi: 10.1038/ncomms8175 (2015).